Mucosal vaccination with attenuatedMycobacterium tuberculosisinduces strong central memory responses and protects against tuberculosis Tuberculosis (TB) is a global pandaemic, partially due to the failure of vaccination approaches. Novel anti-TB vaccines are therefore urgently required. Here we show that aerosol immunization of macaques with the Mtb mutant in SigH (MtbΔ sigH ) results in significant recruitment of inducible bronchus-associated lymphoid tissue (iBALT) as well as CD4 + and CD8 + T cells expressing activation and proliferation markers to the lungs. Further, the findings indicate that pulmonary vaccination with MtbΔ sigH elicited strong central memory CD4 + and CD8 + T-cell responses in the lung. Vaccination with MtbΔ sigH results in significant protection against a lethal TB challenge, as evidenced by an approximately three log reduction in bacterial burdens, significantly diminished clinical manifestations and granulomatous pathology and characterized by the presence of profound iBALT. This highly protective response is virtually absent in unvaccinated and BCG-vaccinated animals after challenge. These results suggest that future TB vaccine candidates can be developed on the basis of MtbΔ sigH . Despite widespread use of the bacille Calmette-Guérin (BCG) vaccine, Mycobacterium tuberculosis ( Mtb ) infection and the resulting incidence of tuberculosis (TB) remains a major global concern. The BCG vaccine, to a large extent and with some exceptions, mitigates only the most severe aspects of infection and exhibits a highly variable efficacy, especially in high-burden areas [1] . The majority of Mtb -infected individuals, including BCG-vaccinated ones, develop persistent but asymptomatic TB infection following Mtb exposure, rather than sterilizing immunity [2] . These individuals retain a finite risk of reactivation because of comorbidities such as HIV or diabetes. Developing new and efficacious TB vaccines is clearly the most effective intervention for containing the TB pandaemic [3] , [4] , [5] . To this end, a number of novel candidates are currently being evaluated either as potential replacements for BCG or to boost BCG-generated responses using a variety of approaches [6] . However, a frontline candidate that attempted to boost existing BCG responses failed to protect a target population against TB in a high-burden setting [7] . These results provide further impetus to the objective of replacing BCG with a new live attenuated vaccine. The failure to generate an effective TB vaccine is attributed to a lack of specific immune correlates of protection from Mtb infection and TB disease. Of interest are adaptive responses, particularly pathogen-specific memory CD4 + and CD8 + T-cell-mediated responses essential for successful bacterial control during LTBI. BCG is generally considered to be inefficient in generating central memory CD4 + and CD8 + T-cell responses [8] , although long-term immunity following BCG administration is possible in some settings [9] . This contributes to the widely perceived inability of the vaccine to confer long-term protection against TB [10] . Thus, understanding related immune parameters and how perturbation by comorbidities leads to TB may be useful for effective TB vaccine design. Aerosol delivery of BCG to the lung enhances protective efficacy [11] , including in macaques [12] . Further, aerosol TB vaccination might allow co-delivery of vaccine and adjuvants [13] . Aerosol–BCG resulted in significantly improved protection in guinea pigs against Mtb challenge compared with conventional vaccination [11] . Besides, an adenoviral vector expressing Mtb antigens elicited robust responses following aerosol delivery [14] . Attenuated mycobacteria have evoked interest as potential BCG-replacement vaccines [15] . The Mtb antigen repertoire counterintuitively evokes strong immunity, suggesting that such responses work in the pathogen’s favour [16] . Immune-evasive pathways of Mtb are therefore the key to understand mechanisms of Mtb persistence [17] . SigH orchestrates a key stress-response pathway in Mtb that mitigates oxidative stress through induction of antioxidant production [18] . The Mtb mutant in sigE , which is part of the SigH regulon, elicited protection from Mtb infection [19] . Further, the M. avium paratuberculosis sigH mutant is being evaluated as a candidate vaccine for protecting cattle (US20140271719A1 (Pending US Patent, Adel Talaat)). Besides, aerosol immunization of macaques with the MtbΔ sigH mutant failed to cause disease [20] . This was in direct contrast to the phenotype of this mutant in C57Bl/6 mice, in which the sigH -null strain replicated to levels comparable to those of parental Mtb [18] . While the MtbΔ sigH mutant in H37Rv did not have a phenotype in monocytes [21] , the mutant in the CDC1551 strain exhibited growth restriction in bone marrow-derived macrophages (BMDMs) [22] . These results suggest that MtbΔ sigH fails to neutralize host-generated oxidants in vivo and is controlled in an elite manner by the primate innate immune system. Macaques accurately model several aspects of the human TB syndrome including partial protection from BCG vaccination [23] , [24] , different outcomes [25] and the full spectrum of pathology [26] , and have the unique capacity to model Mtb /HIV co-infection [28] , [29] . A World Health Organization working group strongly recommended validation of candidate live TB vaccines in this model [30] . In the current study, aerosol vaccination with MtbΔ sigH elicited strong CD4 + and CD8 + central memory T-cell responses as well as a robust T-helper 1 (Th1) response correlating with significantly greater protection from lethal Mtb challenge in rhesus macaques. Furthermore, protection from lethal TB in MtbΔ sigH -vaccinated animals was characterized by the presence of highly organized bronchus-associated lymphoid tissue (iBALT) associated with granulomas, following Mtb challenge. MtbΔ sigH infection and increased iBALT We have previously established a correlation between the levels of ectopic lymphoid structures known as iBALT and the control of Mtb infection in a latent state. Experimentally infected macaques had significantly greater levels of iBALT in their lungs during LTBI, and this response was markedly reduced during TB disease [31] . iBALT was characterized by the presence of CD20 + B and CXCR5 + T cells. The expression of CXCR5 on T cells within iBALT follicles governed correct orientation and localization of T cells and macrophage activation [31] . Since aerosol infection of macaque lungs with MtbΔ sigH resulted in the virtually complete clearance of infection, we used samples from this previous study [20] to assess whether the lungs of MtbΔ sigH -infected macaques harboured increased iBALT. Lung sections from six macaques, each exposed to high doses of Mtb CDC1551 strain or the isogenic MtbΔ sigH mutant, were co-stained for expression of CD3 and CD45R (B220) [31] . Immunofluorescence revealed that lung lesions from animals infected with the mutant contained significantly greater iBALT signal ( Fig. 1a ), relative to those infected with Mtb ( Fig. 1b ). The percentage of area occupied by iBALT was significantly greater in samples from MtbΔ sigH -infected than Mtb -infected animals ( P <0.05; Fig. 1c ). In addition, the total lung area involved in iBALT follicles (μm 2 ; P <0.01) and the average size of these iBALT follicles (μm 2 ; P <0.0001, Student’s t -test) was also significantly greater in sections derived from MtbΔ sigH -infected, relative to Mtb -infected animals ( Supplementary Fig. 1a,b ). These results further support our previous observations that protection from Mtb infection directly correlates with the presence of granuloma-associated iBALT and suggested that the lungs of MtbΔ sigH -infected macaques could exemplify an environment conducive to protection from TB. 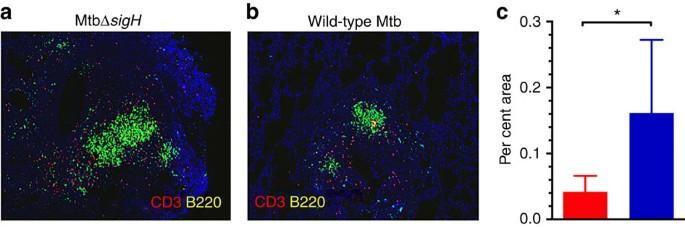Figure 1: iBALT formation induced by MtbΔsigHvaccination. Co-staining with CD3 and B220 revealed that lung granulomas following infection with MtbΔsigH(a) exhibited a significantly increased iBALT response relative to infection withMtb(b). White scale bar, 500 μm. Data from multiple lesions from six different animals were used in the analyses. (c) The percentage of area occupied by iBALT follicles relative to total lung area was analysed in animals challenged withMtb(red) and MtbΔsigH(dark blue). *P<0.05 (Student’st-test). Data are means±s.d. Samples from four to five animals in each group were used for analysis. Figure 1: iBALT formation induced by MtbΔ sigH vaccination. Co-staining with CD3 and B220 revealed that lung granulomas following infection with MtbΔ sigH ( a ) exhibited a significantly increased iBALT response relative to infection with Mtb ( b ). White scale bar, 500 μm. Data from multiple lesions from six different animals were used in the analyses. ( c ) The percentage of area occupied by iBALT follicles relative to total lung area was analysed in animals challenged with Mtb (red) and MtbΔ sigH (dark blue). * P <0.05 (Student’s t -test). Data are means±s.d. Samples from four to five animals in each group were used for analysis. Full size image Analysis of aerosol-MtbΔ sigH as an anti-TB vaccine candidate Encouraged by the magnitude of iBALT induction in macaques infected with MtbΔ sigH , we conceived a vaccine study to assess both the immunogenicity as well as the efficacy of this mutant as a potential vaccine against pulmonary TB. The design of the macaque study is outlined in Fig. 2a . Since enhanced iBALT responses were observed in the lungs of animals infected with the mutant strain via the aerosol route, we postulated that vaccination via the same route would have a greater chance of eliciting protection. Furthermore, BCG vaccination is more effective via the pulmonary route, indicating that local responses, elicited by matching the route of the vaccination to that of infection, may be critical to protect against TB [11] , [12] . Before and following single aerosol vaccination with MtbΔ sigH at a dose that elicited strong iBALT response [20] , both peripheral blood and lung compartments were repeatedly sampled to obtain cells for immune studies and transcriptomics. Eight weeks post vaccination, animals were challenged via aerosol, with a highly lethal dose of Mtb . Unvaccinated and BCG (aerosol)-vaccinated groups were included as appropriate controls ( Fig. 2a ). All animals that received aerosol–BCG or MtbΔ sigH vaccination became tuberculin skin test (TST) positive ( Supplementary Table 1 ). 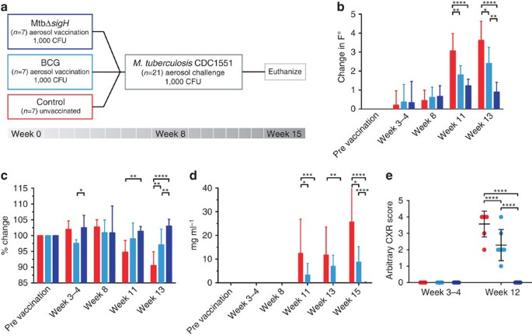Figure 2: Study outline and clinical correlates of vaccination and infection. (a) Three groups of seven macaques were used: unvaccinated (red); vaccinated with BCG (light blue) and vaccinated with MtbΔsigH(dark blue). (b) Changes (Δ°F) in body temperature; (c) changes in percentage of body weight; (d) changes in serum CRP (μg ml−1) levels; and (e) changes in relative thoracic radiograph (CXR) scores, over the course of the vaccination and infection phases. CXRs were scored in a blinded manner by categorizing between zero and four based on increasing involvement in the granulomatous pathology. *P<0.05, **P<0.01, ***P<0.001, ****P<0.0001 using two-way ANOVA with Tukey’s correction for multiple comparisons. Data are means±s.d. Samples from all seven animals in each group were used for analysis at each time point. Figure 2: Study outline and clinical correlates of vaccination and infection. ( a ) Three groups of seven macaques were used: unvaccinated (red); vaccinated with BCG (light blue) and vaccinated with MtbΔ sigH (dark blue). ( b ) Changes (Δ°F) in body temperature; ( c ) changes in percentage of body weight; ( d ) changes in serum CRP (μg ml −1 ) levels; and ( e ) changes in relative thoracic radiograph (CXR) scores, over the course of the vaccination and infection phases. CXRs were scored in a blinded manner by categorizing between zero and four based on increasing involvement in the granulomatous pathology. * P <0.05, ** P <0.01, *** P <0.001, **** P <0.0001 using two-way ANOVA with Tukey’s correction for multiple comparisons. Data are means±s.d. Samples from all seven animals in each group were used for analysis at each time point. Full size image Absence of disease on vaccination with MtbΔ sigH or BCG Aerosolization of broth-cultured, log-phase BCG and MtbΔ sigH was performed as described in the Methods section [20] , [25] , [29] , [32] , [33] . Microbial efficiency of BCG and MtbΔ sigH was highly equivalent during aerosolization. Aerosol vaccination of macaques with MtbΔ sigH and BCG deposited ∼ 1,000 colony-forming unit (CFU) bacilli into the deep lung. Aerosol vaccination with either strain resulted in a positive TST ( Supplementary Table 1 ) but did not induce dyspnoea, anorexia or significant changes in body temperatures relative to pre-infection values ( Fig. 2b ). The body weights of all vaccinated animals also remained relatively normal during the post-vaccination/pre-challenge phase with the exception of a slight decline (<3%) in the body weights of BCG-vaccinated animals 3–4 weeks post vaccination ( Fig. 2c ). None of the vaccinated animals exhibited an increase in serum C-reactive protein (CRP) levels relative to unvaccinated animals at any time post vaccination ( Fig. 2d ). Further, thoracic radiographs acquired post vaccination on all 14 vaccinated animals were normal ( Fig. 2e ). Differential persistence of MtbΔ sigH and BCG in BAL The persistence of live mycobacteria was evaluated in bronchoalveolar lavage (BAL) from both MtbΔ sigH - and BCG-vaccinated macaques. Three weeks after vaccination, greater levels of MtbΔ sigH were recovered from BAL compared with BCG ( Fig. 3a ). At week 5 post vaccination, BCG could not be recovered from BAL, while detectable levels of MtbΔ sigH were still recovered ( Fig. 3a ), indicating that this strain might persist longer than BCG in human lungs. Eight weeks after vaccination, CFU for neither strain was recovered from the BAL of vaccinated macaques. Furthermore, macaque BMDMs were able to kill BCG at a faster rate than both Mtb and MtbΔ sigH in vitro ( Fig. 3b ). BMDMs infected with MtbΔ sigH expressed greater levels of tumour-necrosis factor-α (TNF-α) and interleukin (IL)-1β but not IL-6 transcripts relative to BCG ( Fig. 3c ). In addition, BMDMs infected with MtbΔ sigH also secreted significantly lower levels of inflammatory chemokines CXCL9 ( Fig. 3d ) and CXCL10 ( Fig. 3e ) in supernatants, relative to the BCG-vaccinated or the unvaccinated groups. Both the expression and anti- Mtb activity of TNF-α is strongly enhanced by IL-1β via direct augmentation of caspase-dependent apoptosis [34] . Infection of BMDMs with MtbΔ sigH results in both higher TNF-α expression and greater apoptosis relative to Mtb [22] . The activity of IL-1β is itself regulated by Type I interferons, whose expression is positively controlled by IRF1 and negatively by IRF2. Elicitation of Type I interferon response inhibits IL-1β and TNF-α activity, and promotes the progression of active TB, as is the case during infection with hypervirulent Mtb strains [35] . Abrogation of Type I responses reverses this trend and is being considered as a host-directed therapy for TB [36] . Accordingly, the expression of Type I genes was significantly higher in BAL samples obtained 3 weeks after vaccination from animals that received BCG, and significantly lower in animals that received MtbΔ sigH ( Fig. 3f ). The IRF2 gene expression level was lower in the BAL of BCG-vaccinated and more than twofold higher in the BAL of MtbΔ sigH -vaccinated animals ( Fig. 3f ). The expression of prototypical Type I molecule IFN-γ was also higher in BMDMs infected with BCG and Mtb , relative to those infected with MtbΔ sigH ( Fig. 3c ). 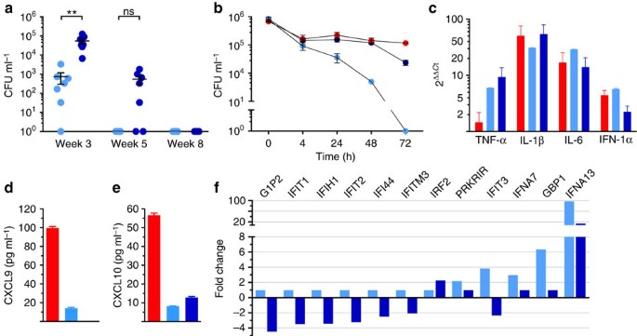Figure 3: Comparative measures of bacterial burden in BAL following aerosol vaccination and restriction during intraphagosomal culturingin vitro. (a) BCG (light blue) and MtbΔsigH(dark blue) CFU levels in total BAL samples at weeks 3, 5 and 8 after vaccination. (b) Rhesus macaque BMDMin vitrokilling assay in CFU ml−1withMtb(red), BCG and MtbΔsigH. **P<0.01 using two-way ANOVA with Tukey’s correction for multiple comparisons. Data are means±s.d. (c) Relative expression (2ΔΔCt) of TNF-α, IL-1β, IL-6 and IFN-1α in BMDMs infected withMtb, BCG and MtbΔsigHusing real-time RT–PCR. (d,e) Absolute expression of CXCL9 (d) and CXCL10 (e; pg ml−1) in supernatants derived from BMDMs infected withMtb, BCG and MtbΔsigHusing cytokine analysis assay. (f) Microarray-derived fold changes of gene expression of 12 Type I interferon genes in the BAL of BCG- and MtbΔsigH-vaccinated animals. For analysis involving BAL, samples from all seven animals in each group were used for analysis at each time point (a). For CFU analysisin vitro, the experiment was performed twice, with four biological replicates in each instance (b). Transcript and cytokine analyses were performed on biological replicates (c–f). ns, not significant. Figure 3: Comparative measures of bacterial burden in BAL following aerosol vaccination and restriction during intraphagosomal culturing in vitro . ( a ) BCG (light blue) and MtbΔ sigH (dark blue) CFU levels in total BAL samples at weeks 3, 5 and 8 after vaccination. ( b ) Rhesus macaque BMDM in vitro killing assay in CFU ml −1 with Mtb (red), BCG and MtbΔ sigH . ** P <0.01 using two-way ANOVA with Tukey’s correction for multiple comparisons. Data are means±s.d. ( c ) Relative expression (2 ΔΔ C t ) of TNF-α, IL-1β, IL-6 and IFN-1α in BMDMs infected with Mtb , BCG and MtbΔ sigH using real-time RT–PCR. ( d , e ) Absolute expression of CXCL9 ( d ) and CXCL10 ( e ; pg ml −1 ) in supernatants derived from BMDMs infected with Mtb , BCG and MtbΔ sigH using cytokine analysis assay. ( f ) Microarray-derived fold changes of gene expression of 12 Type I interferon genes in the BAL of BCG- and MtbΔ sigH -vaccinated animals. For analysis involving BAL, samples from all seven animals in each group were used for analysis at each time point ( a ). For CFU analysis in vitro , the experiment was performed twice, with four biological replicates in each instance ( b ). Transcript and cytokine analyses were performed on biological replicates ( c – f ). ns, not significant. Full size image MtbΔ sigH induces protective immune signatures in the lung Global immune responses to vaccination with MtbΔ sigH or BCG were analysed by transcriptome profiling of BAL samples collected before vaccination and 3 weeks post vaccination. The genes significantly induced in BAL after BCG vaccination were involved in cellular transport, DNA binding by regulatory protein, RNA processing or were part of the lumen, non-membrane-bound organelle or macromolecular complex assembly ( Fig. 4 ). The only major category of genes induced following BCG vaccination was that categorized as pertaining to immune system development ( Fig. 4 ). Conversely, the expression of genes involved in NK cell signalling, MAPK signalling and JAK/STAT signalling, cytokine signalling, T-cell signalling, calcium signalling, neuroactive/growth receptors and lipid biosynthesis were induced to higher levels in the BAL from MtbΔ sigH -vaccinated macaques ( Fig. 4 ). Further, a large majority of these genes were either not expressed or were expressed to significantly lower levels in the BAL of animals vaccinated with BCG ( Fig. 4 ). Thus, vaccination with MtbΔ sigH appeared to result in the induction of a markedly stronger innate immune response, as indicated by the differential induction of NK cell, MAPK and JAK/STAT signalling pathways as well as genes from the cytokine, T-cell receptor and calcium signalling pathways ( Fig. 4 ), although the differential persistence of the two mycobacterial strains could have played a role in this differential response. In addition, enhanced immune cell differentiation, proliferation, activation and processing, as well as macromolecular synthesis, which are associated with heightened cytokine and T-cell responses, were evidenced by the increased expression levels of neuroactive/growth factor receptor signalling, potentiation and lipid biosynthesis pathways in BAL samples derived from animals vaccinated with MtbΔ sigH ( Fig. 4 ). 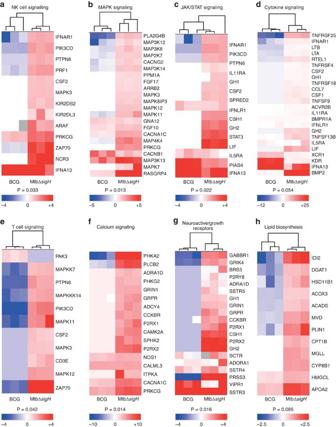Figure 4: Transcriptomics from BAL 3 weeks after immunization. Total RNA isolated from BAL samples of three animals vaccinated with BCG and another three with MtbΔsigH, obtained 3 weeks after vaccination, was subjected to amplification and macaque-specific DNA microarray analysis. The expression of genes belonging to natural killer cells (a), MAP Kinase (b), JAK/STAT (c), cytokine (d), T cells (e), calcium signalling (f), neuroactive/growth receptors (g) and lipid biosynthesis (h) pathways were induced to significantly higher levels in the BAL of animals vaccinated with MtbΔsigH, relative to those vaccinated with BCG.Pvalues shown are derived from the analysis of significant terms in DAVID with Bonferroni correction for multiple comparisons. BAL samples from three animals in each group were used for microarray experiments. Figure 4: Transcriptomics from BAL 3 weeks after immunization. Total RNA isolated from BAL samples of three animals vaccinated with BCG and another three with MtbΔ sigH , obtained 3 weeks after vaccination, was subjected to amplification and macaque-specific DNA microarray analysis. The expression of genes belonging to natural killer cells ( a ), MAP Kinase ( b ), JAK/STAT ( c ), cytokine ( d ), T cells ( e ), calcium signalling ( f ), neuroactive/growth receptors ( g ) and lipid biosynthesis ( h ) pathways were induced to significantly higher levels in the BAL of animals vaccinated with MtbΔ sigH , relative to those vaccinated with BCG. P values shown are derived from the analysis of significant terms in DAVID with Bonferroni correction for multiple comparisons. BAL samples from three animals in each group were used for microarray experiments. Full size image Local increases in T cells due to MtbΔ sigH vaccination Local and systemic immune responses were compared following vaccination by analysis of BAL and blood, respectively. Marked increases in CD4 + and CD8 + T-cell numbers were found in BAL immediately post vaccination ( P <0.001; two-way analysis of variance analysis of variance (ANOVA) with Tukey’s correction; Fig. 5a,b ); however, no differences in the frequency of CD4 + and CD8 + T cells were observed in the periphery post vaccination ( Supplementary Fig. 2 ). In addition, no differences in the chemokine receptors CXCR3, CXCR4, CCR7 or activation marker CD69 were detected systemically, which indicated no significant variation in the functional phenotype of T cells in the blood ( Supplementary Fig. 3 ). However, a significant increase in the number of circulating CD4 + CCR5 + T cells was discovered in the MtbΔ sigH group between weeks 2 and 3 ( P <0.05; two-way ANOVA with Tukey’s correction; Supplementary Fig. 3 ). No differences were observed in the memory status of circulating T cells, including central (T CM− CD28 + CD95 + ) and effector memory (T EM− CD28 − CD95 + ) cells or naïve T cells (CD28 + CD95 − ; Supplementary Fig. 2 ) [37] . 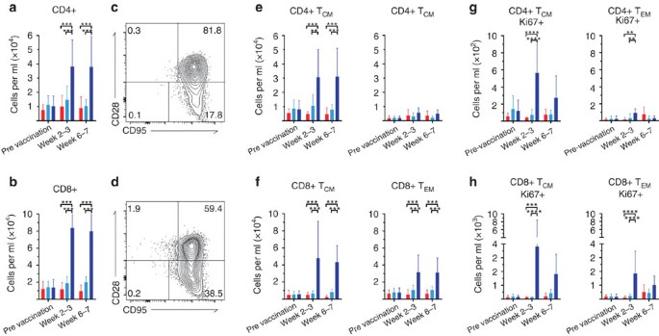Figure 5: T-cell response to immunization in BAL. Vaccination with MtbΔsigH(dark blue) induced a significantly higher central memory immune response relative to BCG vaccination (light blue), or no vaccination (red). Quantification of CD4+(a) and CD8+(b) T cells migrating to the lung after vaccination. Representative plots of central memory (CD28+CD95+), effector memory (CD28−CD95+) and naive (CD28+CD95−) CD4+(c,e) and CD8+(d,f) T cells in BAL. Quantification of CD4+(e) TCMand TEMcells, CD8+TCMand TEMcells (f) in BAL, and the proliferative capability of these cells (g,h). *P<0.05; **P<0.01; ***P<0.001; ****P<0.0001 using two-way ANOVA with Tukey’s correction for multiple comparisons. Data are means±s.d. BAL samples from all 21 animals (n=7, three groups) were included in the flow cytometry experiments and analyses. Samples from all seven animals in each group were used for analysis at each time point. Figure 5: T-cell response to immunization in BAL. Vaccination with MtbΔ sigH (dark blue) induced a significantly higher central memory immune response relative to BCG vaccination (light blue), or no vaccination (red). Quantification of CD4 + ( a ) and CD8 + ( b ) T cells migrating to the lung after vaccination. Representative plots of central memory (CD28 + CD95 + ), effector memory (CD28 − CD95 + ) and naive (CD28 + CD95 − ) CD4 + ( c , e ) and CD8 + ( d , f ) T cells in BAL. Quantification of CD4 + ( e ) T CM and T EM cells, CD8 + T CM and T EM cells ( f ) in BAL, and the proliferative capability of these cells ( g , h ). * P <0.05; ** P <0.01; *** P <0.001; **** P <0.0001 using two-way ANOVA with Tukey’s correction for multiple comparisons. Data are means±s.d. BAL samples from all 21 animals ( n =7, three groups) were included in the flow cytometry experiments and analyses. Samples from all seven animals in each group were used for analysis at each time point. Full size image While no significant changes were discovered in T-cell frequencies in the peripheral blood, a strong lung-specific central and effector memory response was initiated post vaccination with MtbΔ sigH . This response was apparent immediately after vaccination by significant increases in the number of CD4 + central memory (T CM ) ( P <0.01–0.001; two-way ANOVA with Tukey’s correction) as well as CD8 + T CM and effector memory (T EM ; P <0.001) in the BAL ( Fig. 5c–f ), with a marked increase in proliferation as measured by Ki67 positivity ( P <0.01–0.0001; Fig. 5g,h ). A significant increase in the number of CD69 + T cells ( P <0.001 for MtbΔ sigH versus BCG and P <0.01–0.001 for MtbΔ sigH versus unvaccinated groups; Fig. 6a,b ) indicated that T cells in BAL were antigen-stimulated via the T-cell receptor. The polarity of the T-cell response was examined using the markers CCR5 and CXCR3, which are preferentially expressed by Th1 cells, as well as CXCR4, which is preferentially expressed by T-helper 2 (Th2) cells. The results revealed that T cells in BAL immediately post-MtbΔ sigH vaccination preferentially expressed high levels of CCR5 and CXCR3 compared with T cells recruited following vaccination with BCG ( P <0.01–0.001; Fig. 6c,d ). Thus, aerosol vaccination with MtbΔ sigH induced transcriptomic and cellular signatures indicative of a strong Th1 response that resulted in accumulation of memory T cells. 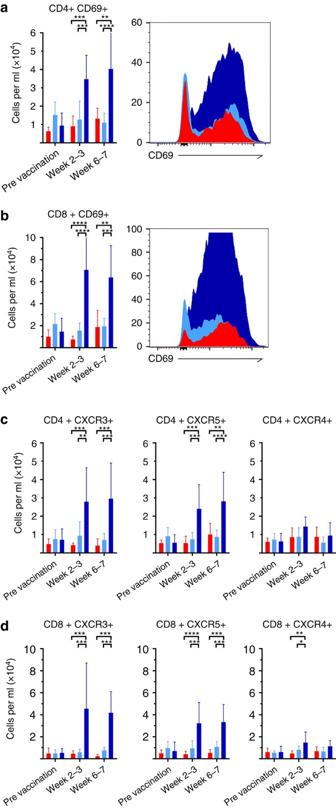Figure 6: Local T-cell phenotype to immunization in BAL. Vaccination with MtbΔsigH(dark blue) induced a significantly stronger TH1 cell response relative to BCG vaccination (light blue), or no vaccination (red). Quantification of and representative histograms of CD4+CD69+(a) and CD8+CD69+(b) T cells migrating to the lung after vaccination. Absolute cell counts of phenotypic markers CXCR3, CCR5 and CXCR4 in CD4+(c) and CD8+(d) T cells in BAL at different stages of infection. *P<0.05, **P<0.01, ***P<0.001, ****P<0.0001 using two-way ANOVA with Tukey’s correction for multiple comparisons. Data are means±s.d. BAL samples from all 21 animals (n=7, three groups) were included in the flow cytometry experiments and analyses. Samples from all seven animals in each group were used for analysis at each time point. Figure 6: Local T-cell phenotype to immunization in BAL. Vaccination with MtbΔ sigH (dark blue) induced a significantly stronger T H 1 cell response relative to BCG vaccination (light blue), or no vaccination (red). Quantification of and representative histograms of CD4 + CD69 + ( a ) and CD8 + CD69 + ( b ) T cells migrating to the lung after vaccination. Absolute cell counts of phenotypic markers CXCR3, CCR5 and CXCR4 in CD4 + ( c ) and CD8 + ( d ) T cells in BAL at different stages of infection. * P <0.05, ** P <0.01, *** P <0.001, **** P <0.0001 using two-way ANOVA with Tukey’s correction for multiple comparisons. Data are means±s.d. BAL samples from all 21 animals ( n =7, three groups) were included in the flow cytometry experiments and analyses. Samples from all seven animals in each group were used for analysis at each time point. Full size image Vaccination with MtbΔ sigH protects from lethal Mtb challenge To evaluate the potential of the attenuated mycobacterium to serve as a TB vaccine, all animals were challenged with a high dose of Mtb CDC1551, which has historically produced lethal TB in rhesus macaques within 10 weeks [20] , [32] . Unvaccinated animals rapidly developed pulmonary granulomatous pathology with rapid increases in body temperatures ( P <0.01 for MtbΔ sigH relative to BCG and P <0.0001 for MtbΔ sigH versus unvaccinated groups; two-way ANOVA with Tukey’s correction) and serum CRP levels ( P <0.0001 for MtbΔ sigH versus both other groups; Fig. 2b,d ), as well as a swift decline in body weights P <0.01 for MtbΔ sigH relative to BCG and P <0.0001 for MtbΔ sigH versus unvaccinated groups; Fig. 2c ). Control animals also exhibited high levels of pulmonary granulomatous involvement by radiology ( Fig. 2e ). The same clinical measure also increased, albeit to a lesser degree, in animals that were aerosol-vaccinated with BCG, while animals vaccinated with MtbΔ sigH exhibited virtually no evidence of disease ( P <0.0001 for MtbΔ sigH versus unvaccinated as well as versus BCG; Fig. 2b–e ). Three weeks post- Mtb challenge (week 11), the increase in body temperatures in unvaccinated animals was significant relative to BCG-vaccinated ( P <0.01) and highly significant relative to MtbΔ sigH -vaccinated animals ( P <0.0001; two-way ANOVA with Tukey’s correction; Fig. 2b ). Five weeks post challenge (week 13), the differences in body temperature between the unvaccinated and BCG-vaccinated groups were significant ( P <0.05); the differences between the BCG and MtbΔ sigH -vaccinated groups were very significant ( P <0.01); and the differences between the unvaccinated and MtbΔ sigH -vaccinated groups were highly significant ( P <0.0001; Fig. 2b ). The differences in body weight between the unvaccinated and MtbΔ sigH -vaccinated groups and the BCG and MtbΔ sigH -vaccinated groups were very significant at week 11 ( P <0.01; Fig. 2c ) and while by week 13, these differences had become highly significant ( P <0.0001; two-way ANOVA with Tukey’s correction). Profoundly lower serum CRP levels were detected in the macaques vaccinated with MtbΔ sigH relative to macaques that were not vaccinated at weeks 11 and 13 and at time of euthanasia ( P <0.0001). At both week 11 ( P <0.05) and while euthanasia ( P <0.0001; two-way ANOVA with Tukey’s correction), the serum CRP levels detected in the macaques vaccinated with MtbΔ sigH were also significantly lower than levels measured in the BCG-vaccinated group ( Fig. 2d ). Similarly, animals vaccinated with MtbΔ sigH exhibited significantly lower chest X-ray (CXR) scores, consistent with lack of disease following lethal challenge, in this group, relative to either BCG-vaccinated or unvaccinated macaques ( P <0.0001 in both cases). While extensive pathology was not discernable in the lungs of macaques vaccinated with the mutant, a majority of those vaccinated with BCG exhibited moderate CXR scores, again significantly lower than those in the unvaccinated group, where pathology consistent with military TB could be observed in a majority of animals. Vaccination with MtbΔ sigH reduces in vivo bacterial burdens The protection conferred by MtbΔ sigH was also evident following evaluation of bacterial burdens. Significantly lower Mtb was recovered from BAL from MtbΔ sigH -vaccinated animals relative to those vaccinated with BCG at 3 and 5 weeks after challenge (weeks 11 and 13; Fig. 7a ). At the time of euthanasia, the total lung burden in animals vaccinated with MtbΔ sigH was three logs lower than burdens in unvaccinated ( P <0.01) and two logs lower than burdens in BCG-vaccinated ( P <0.01) animals, while bacterial loads in animals vaccinated with BCG were only 0.5–1 logs lower than in the control group ( P <0.05; one-way ANOVA with Tukey’s correction; Fig. 7b ). We were unable to culture Mtb from >42% of all lung sections obtained from macaques vaccinated with MtbΔ sigH . In contrast, every section obtained from either unvaccinated animals or those vaccinated with BCG was positive for Mtb . Thus, the Mtb burden was significantly lower in the lungs of MtbΔ sigH -vaccinated animals following lethal challenge compared with those vaccinated with BCG. Similar results were obtained when bronchial lymph node bacterial burdens were analysed at necropsy ( Fig. 7c ). Using a combination of hygromycin resistance/sensitivity and PCR, we verified that the obtained CFUs were Mtb and not residual MtbΔ sigH or BCG. 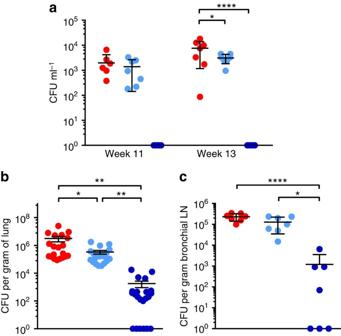Figure 7: Bacterial burden following lethalMtbchallenge. (a)MtbCFU levels in total BAL samples at week 11 (3 weeks after challenge) and week 13 (5 weeks after challenge; (b).Mtblevels per gram of lung tissue at necropsy (c).Mtbburdens per gram of bronchial lymph node tissue at *P<0.05; **P<0.01; ***P<0.001; ****P<0.0001, (a) two-way ANOVA and (b,c) one-way ANOVA with Tukey’s multiple testing correction. Data are means±s.d. Samples from all seven animals in each group were used for analysis at each time point. For analysis of lung burdens, four pooled samples (two each from left and right lung) from each macaque, each representing five distinct lung sections were used (b). For analysis of bronchial lymph node burdens, one section from each animal was analysed. Figure 7: Bacterial burden following lethal Mtb challenge. ( a ) Mtb CFU levels in total BAL samples at week 11 (3 weeks after challenge) and week 13 (5 weeks after challenge; ( b ). Mtb levels per gram of lung tissue at necropsy ( c ). Mtb burdens per gram of bronchial lymph node tissue at * P <0.05; ** P <0.01; *** P <0.001; **** P <0.0001, ( a ) two-way ANOVA and ( b , c ) one-way ANOVA with Tukey’s multiple testing correction. Data are means±s.d. Samples from all seven animals in each group were used for analysis at each time point. For analysis of lung burdens, four pooled samples (two each from left and right lung) from each macaque, each representing five distinct lung sections were used ( b ). For analysis of bronchial lymph node burdens, one section from each animal was analysed. Full size image Vaccination with MtbΔ sigH leads to reduced lung pathology The results of the pulmonary pathology analyses mirrored those obtained following analysis of bacterial burdens. Animals vaccinated with MtbΔ sigH exhibited significantly fewer pulmonary lesions on challenge, as determined by both gross and histopathological examination ( Fig. 8a–f and Supplementary Fig. 4 ) and morphometric quantitation ( Fig. 8g ). Thus, the animals vaccinated with MtbΔ sigH had fewer granulomas (the extent of lung affected by TB lesions following Mtb infection encompassed an average of 4%), and less TB-related pathology (for example, oedema, pneumonia and generalized foci of inflammation) than animals in the other two groups (where ∼ 40% of the lung was affected; P <0.0001 in both cases; one-way ANOVA with Tukey’s correction; Fig. 8g ). The clinical and microbiological differences also correlated with significant differences in overall survival rates following challenge ( Fig. 8h ). All seven unvaccinated animals succumbed to massive pulmonary TB following a lethal aerosol Mtb challenge within a median of 36 days. Five out of seven BCG-vaccinated animals also succumbed to TB, within a median of 48 days. None of the MtbΔ sigH -vaccinated animals exhibited any overt signs of disease or required euthanasia ( Fig. 8h ). 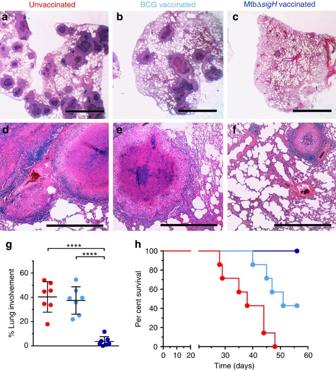Figure 8: Histopathological and survival analysis of lungs ofMtb-infected animals. Haematoxylin and eosin (H&E) staining from representative animals in each of the three groups. (a,d) Vaccine-naive group with miliary, white 2–4 mm granulomas and scattered lobular multicoloured areas of consolidation. (b,e) BCG-vaccinated with localized dark red lobar pneumonia and (c,f) MtbΔsigH-vaccinated with no apparent gross lesions. Black scale bars in (a–c), 5 mm and (d–f), 500 μm. (g) Morphometric measures of pulmonary pathology in the different groups of unvaccinated (red), BCG-vaccinated (light blue) and MtbΔsigH-vaccinated (dark blue) animals. ****P<0.0001 with (g) one-way ANOVA using Tukey’s multiple testing correction. Data are means±s.d. (h) Survival proportion Kaplan–Meier curves for the three groups of animals, using Mantel–Cox (log-rank) survival analysis. At least three systematic random microscopic fields from each lung, representing most lung lobes, from each of the animals in every group were used for morphometric analysis (g). Data from each of the seven animals per group was used for survival proportions analysis (h). Figure 8: Histopathological and survival analysis of lungs of Mtb -infected animals. Haematoxylin and eosin (H&E) staining from representative animals in each of the three groups. ( a , d ) Vaccine-naive group with miliary, white 2–4 mm granulomas and scattered lobular multicoloured areas of consolidation. ( b , e ) BCG-vaccinated with localized dark red lobar pneumonia and ( c , f ) MtbΔ sigH -vaccinated with no apparent gross lesions. Black scale bars in ( a – c ), 5 mm and ( d – f ), 500 μm. ( g ) Morphometric measures of pulmonary pathology in the different groups of unvaccinated (red), BCG-vaccinated (light blue) and MtbΔ sigH -vaccinated (dark blue) animals. **** P <0.0001 with ( g ) one-way ANOVA using Tukey’s multiple testing correction. Data are means±s.d. ( h ) Survival proportion Kaplan–Meier curves for the three groups of animals, using Mantel–Cox (log-rank) survival analysis. At least three systematic random microscopic fields from each lung, representing most lung lobes, from each of the animals in every group were used for morphometric analysis ( g ). Data from each of the seven animals per group was used for survival proportions analysis ( h ). Full size image Differential T-cell responses in animals post challenge To assess an immunologic basis for protection induced by MtbΔ sigH , the functional phenotype of circulating CD4 + and CD8 + T cells was analysed by employing the same markers used for evaluating pulmonary responses following vaccination. No significant differences in the percentages of CD4 + and CD8 + central or effector memory cells were observed in peripheral blood immediately following challenge ( Supplementary Fig. 2 ). However, a significant increase in CD4 + CCR5 + T cells was identified 7 weeks after Mtb challenge, as well as a significant decrease in CD8 + CXCR3 + T cells in peripheral blood at weeks 3 and 7 following challenge in unvaccinated animals ( Supplementary Fig. 3 ). Consistent with overall lung involvement and chest radiograph scores, a significantly greater number of CD4 + and CD8 + T cells including T CM and T EM were present in BAL in the unvaccinated animals compared with both BCG and MtbΔ sigH -vaccinated animals ( Fig. 9a–d ). The increased numbers of T cells in BAL in unvaccinated animals were also evident from representative histograms of CD69 + T cells ( Supplementary Fig. 5a,b ). While no significant differences were observed in CXCR3, CCR5 and CXCR4 expression by CD4 + or CD8 + T cells between the two vaccinated groups ( Supplementary Fig. 5c,d ), a significant decrease in the number of CD8 + CXCR4 + was noted at weeks 11 and 15 in the MtbΔ sigH -vaccinated group compared with the other two groups ( Supplementary Fig. 5d ). 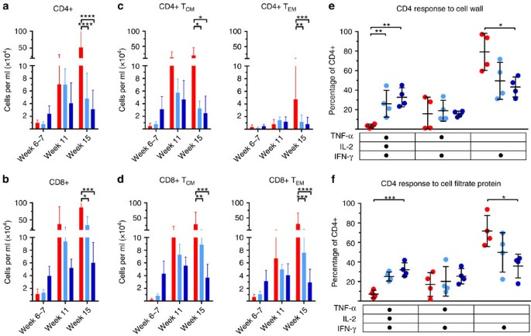Figure 9: Immune responses in the lung post-Mtbchallenge. (a,b) Quantification of cells per ml of BAL of (a) CD4+and (b) CD8+T cells and of (c) CD4+TCMand TEMcells and of (d) CD8+TCMand TEMcells migrating to the lung after challenge in groups of unvaccinated (red), BCG-vaccinated (light blue) and MtbΔsigH-vaccinated (dark blue) animals. (e,f) Percentage of CD4 T cells from PBMCs prepared from whole blood, producing gamma interferon, interleukin 2 and tumour necrosis factor alpha in response to (e) theMtbcell wall and to (f)Mtbcell filtrate protein. *P<0.05, **P<0.01, ***P<0.001, ****P<0.0001 using two-way ANOVA with Tukey’s correction for multiple comparisons. Data are means±s.d. BAL samples from all 21 animals (n=7, three groups) were included in the flow cytometry experiments and analyses (a–d). For antigen-specific studies, samples from four animals per group were employed (e–d). Figure 9: Immune responses in the lung post- Mtb challenge. ( a , b ) Quantification of cells per ml of BAL of ( a ) CD4 + and ( b ) CD8 + T cells and of ( c ) CD4 + T CM and T EM cells and of ( d ) CD8 + T CM and T EM cells migrating to the lung after challenge in groups of unvaccinated (red), BCG-vaccinated (light blue) and MtbΔ sigH -vaccinated (dark blue) animals. ( e , f ) Percentage of CD4 T cells from PBMCs prepared from whole blood, producing gamma interferon, interleukin 2 and tumour necrosis factor alpha in response to ( e ) the Mtb cell wall and to ( f ) Mtb cell filtrate protein. * P <0.05, ** P <0.01, *** P <0.001, **** P <0.0001 using two-way ANOVA with Tukey’s correction for multiple comparisons. Data are means±s.d. BAL samples from all 21 animals ( n =7, three groups) were included in the flow cytometry experiments and analyses ( a – d ). For antigen-specific studies, samples from four animals per group were employed ( e – d ). Full size image Comparison of polyfunctional Mtb -specific T-cell responses To examine antigen-specific responses to Mtb , isolated peripheral blood mononuclear cells (PBMCs) collected 5 weeks post challenge were stimulated with whole Mtb cell wall and cell filtrate protein, and responses were analysed using intracellular cytokine staining for IFN-γ, IL-2 and TNF-α. The results indicated that vaccination with MtbΔ sigH and BCG correlated with significant increases in the percentage of polyfunctional, IFN-γ + , IL-2 + , TNF-α + CD4 + T cells, whereas unvaccinated animals displayed a significantly greater number percentage of monofunctional CD4 + T cells ( Fig. 9e,f ). Unfortunately, samples from other time points were not available for analysis. Profound iBALT post challenge in MtbΔ sigH -vaccinated animals Lung samples collected after lethal Mtb challenge from unvaccinated ( Fig. 10a,d ), BCG-vaccinated ( Fig. 10b,e ) and MtbΔ sigH -vaccinated ( Fig. 10c,f ) macaques at the time of necropsy were assayed for iBALT by histopathology and immunofluorescence with CD3 and CD20 followed by confocal microscopy and image analysis. We observed that protection in each of these groups of macaques was strongly associated with levels of iBALT. Thus, the few, small granulomas in the lungs of animals vaccinated with MtbΔ sigH and challenged with Mtb were characterized by the presence of multiple well-organized iBALT per lesion ( Fig. 10c ). The presence of the follicles was also apparent in the cognate haematoxylin and eosin stains ( Fig. 10 c,f ). These follicles were, in general, associated with granulomas and appeared to be an outgrowth of the outer lymphocyte-rich layer ( Fig. 10 c,f ). While B cells constituted the majority in these follicles, CD3 + cells were also present ( Fig. 10c ). In contrast to the multiple well-developed iBALT associated with granulomas in MtbΔ sigH -immunized animal, animals from the other groups ( Fig. 10a,b,d,e ) had fewer iBALT that were less well organized. The total area of iBALT in MtbΔ sigH -vaccinated macaques was significantly greater after Mtb challenge ( Fig. 10g ) than in either of the other groups, despite the fact that the area occupied by granulomas in the MtbΔ sigH -vaccinated group was significantly less compared with the other two groups after Mtb challenge ( Fig. 10h ). This further emphasizes the difference in BALT induction and the correlation between iBALT and latent control of Mtb infection. 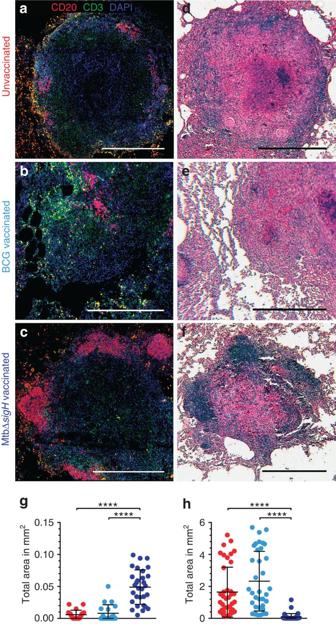Figure 10: Induction of BALT after lethalMtbchallenge correlates with protection from pulmonary granulomatous TB. (a–c) Co-staining of lung sections with CD3 (green) and CD20 (red) and staining of corresponding sections (d–f) with H&E revealed that (a,d) vaccine-naive animals and (b,e) BCG-vaccinated animals had significantly reduced iBALT follicle formation in comparison with (c,f) MtbΔsigH-vaccinated animals, at necropsy, after lethalMtbchallenge. White and black scale bars, 500 μm. Quantification of multiple lesions in six different animals were used the analysis. (g) Total area (mm2) of iBALT follicles and (h) granulomatous pathology in unvaccinated (red), BCG-vaccinated (light blue) and MtbΔsigH-vaccinated (dark blue) animals. ****P<0.0001 using Student’st-test. Data are means±s.d. At least 10 sections from each slide derived from a lung block from multiple animals in each group were used for statistical analysis (g–h). Figure 10: Induction of BALT after lethal Mtb challenge correlates with protection from pulmonary granulomatous TB. ( a – c ) Co-staining of lung sections with CD3 (green) and CD20 (red) and staining of corresponding sections ( d – f ) with H&E revealed that ( a , d ) vaccine-naive animals and ( b , e ) BCG-vaccinated animals had significantly reduced iBALT follicle formation in comparison with ( c , f ) MtbΔ sigH -vaccinated animals, at necropsy, after lethal Mtb challenge. White and black scale bars, 500 μm. Quantification of multiple lesions in six different animals were used the analysis. ( g ) Total area (mm 2 ) of iBALT follicles and ( h ) granulomatous pathology in unvaccinated (red), BCG-vaccinated (light blue) and MtbΔ sigH -vaccinated (dark blue) animals. **** P <0.0001 using Student’s t -test. Data are means±s.d. At least 10 sections from each slide derived from a lung block from multiple animals in each group were used for statistical analysis ( g – h ). Full size image Previously, we showed that aerosolization of a high dose of MtbΔ sigH into the lungs of rhesus macaques resulted in nonpathogenic infection [20] . Here we demonstrate that pulmonary vaccination with this mutant protected against lethal challenge in macaques via the induction of a potent memory T-cell response. Further, we establish a strong correlation between the latent control of infection and iBALT, suggesting that these lymphoid structures facilitate control of TB by maintaining LTBI or sterilizing infection. Induction of BALT in response to respiratory infections is known to not only result in protection, but such responses are also less pathologic [38] . Secondary T FH cells, which constitute the great majority of lymphoid follicle (including iBALT) T cells, expand from memory T cells in a B-cell-aided manner [39] . Our results therefore suggest that the interplay between B and T cells is critical for the proper development of granulomatous-protective responses to TB. This study substantiates previous work using the macaque model of TB, which showed that B cells produced antibody and were important for control of TB [40] . Our results suggest that future studies should unravel the function of B cells recruited to the lung to understand immunity from TB. While the correlates of vaccine-induced protective immunity against TB are not completely understood, T lymphocytes expressing markers of central memory response (dual positivity for CD28 and CD95) [37] are critical for protection. A model of protective immunity that is currently gaining credence suggests that initial vaccination(s) resulting in a spike in effector response can result in the establishment of a central memory response, which is likely to result in long-term protection [41] . T CM are extremely proliferative and can rapidly evolve into large numbers of effector cells expressing high levels of pro-inflammatory cytokines (for example, IFN−γ). Consequently, the finding that pulmonary vaccination with MtbΔ sigH resulted in potent T CM (as well as T EM , particularly CD8 + ) responses during the post-vaccination phase that corresponded to a strong T EM response in the challenge phase merits further evaluation. The role of chemokine receptors, including CXCR3, is critical to the recruitment of CD8 + T cells, and CXCR3 expression on T CM is strongly correlated with effective anti-pathogen memory responses [42] . BAL transcriptome profiling results indicated that animals vaccinated with MtbΔ sigH developed a highly productive pulmonary immune response, both in terms of magnitude and breadth. Prior studies have established that CD4 + T cells with specificity for mycobacterial antigens are critical for the control of Mtb infection [43] , and that CD8 + T cells play an increasingly important role in this process [41] , [44] . SigH induces pathogen antioxidant responses during stress [45] , [46] . MtbΔ sigH is unable to induce expression of the transcriptionally linked thioredoxins and thiol peroxidases [45] that act as antioxidant buffers against the host oxidative burst [47] . Consequently, the antioxidant response of the MtbΔ sigH mutant was strongly crippled [47] , and the resulting production of oxidants likely enhanced antigen-specific CD8 + T-cell responses through the cross-priming of antigen presentation [48] . In addition, the ability of MtbΔ sigH to persist longer than BCG allowed for increased stimulation and antigen presentation, inducing a stronger, more robust, T-cell repertoire [49] . Further characterization of this T CM response is however necessary to substantiate that these cells are not long-lived T EM cells, since MtbΔ sigH antigens persist longer than BCG. The ability of aerosol MtbΔ sigH vaccination to elicit highly protective responses in macaques could have roots in the fundamental processes that govern Mtb –macrophage interactions. In vitro , macrophages infected with this mutant elicited greater expression of Th1 pro-inflammatory cytokines TNF-α and IL-1β, and lower Type I interferon, relative to those infected with Mtb and BCG (this study and ref. 22 ). Together, these results indicate that the interaction of MtbΔ sigH with host phagocytes is critically altered by the loss of the bacillus’s ability to induce SigH-mediated antioxidant functions, relative to BCG. TNF can restrict macrophage-contained Mtb by several mechanisms, including by potently inducing early inflammatory responses [50] , transducing apoptotic signals through activation of caspase 8 (ref. 51 ) activating CD8 cells [52] and potentiating IFN-γ-induced killing of Mtb [53] , [54] . On the other hand, BCG induces strong expression of the SigH regulon (including antioxidants) and is therefore unable to alter these interactions. In fact most BCG strains exhibit duplication of sigH , likely rendering it even less susceptible to phagocyte oxidative mechanisms [55] . In vitro results thus hint at the mechanism by which pulmonary vaccination with MtbΔ sigH could generate protective responses. Unable to counter the host oxidative burst, the mutant elicited greater IL-1β and TNF-α expression leading to significantly greater antimicrobial response, apoptosis and antigen presentation. That Mtb uses Type I signalling to modulate IL-1β expression is well established [56] . CD4 + T cells play a key role in the control of Mtb infection, and polyfunctional cytokine production of antigen-specific Th1 cells is associated with this control [57] . Animals vaccinated with MtbΔ sigH displayed higher frequencies of Mtb cell wall- and culture filtrate protein-responsive polyfunctional CD4 + T cells compared with unvaccinated animals. Recent data have shown that markers of T-cell immune activation in human TB are associated with smear and culture conversion during anti-TB treatment [58] . Nonetheless, the current study had some limitations; for example, protection was only demonstrated in a homologous strain. Thus, future experiments should test the efficacy of the current and related mutants against high-virulence heterologous strains of the same clade as CDC1551, as well as of a different lineage. Second, a lethal challenge at 8 weeks post vaccination may not sufficiently model protection arising from long-term antigen-specific memory T-cell responses. A prior report suggested that BCG failed to induce long-term central memory responses to Mtb infection, which may account for its failure to protect adults against TB [10] . Successful vaccination against TB will require elicitation of both a stable and broad repertoire of memory responses to ensure effective protection against the pathogen during a subsequent infection [41] . While the current results did not establish long-term immunity based on effective elicitation of T CM responses, the findings did demonstrate that prior pulmonary vaccination with MtbΔ sigH resulted in a markedly superior elicitation of both CD4 + and CD8 + T CM responses relative to BCG vaccination. An abundance of data has indicated that T CM lymphocytes retain a potent proliferative capacity and can differentiate into the T EM phenotype when re-exposed to the cognate antigen [59] . The current data demonstrated that MtbΔ sigH elicited a more efficient post-vaccination T CM response, a greater T EM response following challenge and conferred stronger protection. In this study, vaccines were delivered via aerosol, although BCG is given to recipients intradermally. It is impossible to directly compare the results from the aerosol–BCG group to the effectiveness of intradermal BCG vaccination. There have been recent attempts, however, to deliver vaccines, directly to the lung [11] , driven by the pioneering work of Barclay et al . [12] , who showed that macaques could be protected against TB by aerosolized BCG. While a direct comparison of the effectiveness of aerosol-to-intradermal-administered BCG was beyond the scope of this study, preliminary data and prior reports of intradermal BCG vaccination [14] , [24] , [60] suggest that aerosol–BCG outperformed intradermal vaccination in macaques. Although BCG induces potent cellular responses in infants and protects them, neither the responses nor the efficacy are generally considered to be long lasting [61] , although some reports strongly suggest that this is possible [9] . Furthermore, BCG does not completely protect against pulmonary TB including reactivation and reinfection [61] . New vaccines against TB are therefore urgently needed. It has therefore been hypothesized that rationally attenuated strains of Mtb are likely better at serving as vaccine platforms against TB, since these strains are human-adapted, in contrast to bovine-adapted BCG [61] . There are other issues that limit the effectiveness of BCG. It is only able to induce cytokines associated with long-lasting control of Mtb infection several months post vaccination, meanwhile enabling a window of dissemination [62] . Furthermore, Mtb , unlike BCG, retains known immunodominant epitopes for humans. Finally, it has been argued that Mtb expresses genes important for the evasion of host immune responses. SigH is one such gene allowing the pathogen to significantly induce the expression of thioredoxins, which attenuate phagocyte oxidative burst [20] , [22] , [47] . Thus, MtbΔ sigH , a human-adapted strain with a significant immune-evasion impairment, is exceedingly safe even after direct high-dose delivery into primate lungs. In summary, our results provide a roadmap for identifying correlates of protection from TB in a highly human-like model. While it remains to be seen whether such responses can also be elicited following intradermal vaccination, there is considerable renewal of interest in matching the route of vaccination with that of infection in generating protection against TB [13] . Nonhuman primates All animal procedures were approved by the Institutional Animal Care and Use Committee and were performed in strict accordance with the NIH guidelines. Twenty-one specific-pathogen-free, retrovirus-free, mycobacteria-naive, adult rhesus macaques, bred and housed at the Tulane National Primate Research Centre (TNPRC), between the ages of 3 and 12 years were assigned to three groups of seven on the basis of power calculations, which suggested that statistical significance could be detected with sufficient power in these group sizes if addressing a reduction in the average lung bacterial burden by 1log. One group of macaques ( n =7) remained unvaccinated, a second group ( n =7) was vaccinated with a target dose of 1,000 CFU of M. bovis BCG (Danish) while the third group ( n =7) was vaccinated with an equivalent dose of the MtbΔ sigH isogenic mutant in the CDC1551 background. Aerosol vaccination was conducted using the same equipment and procedural configuration as the Mtb challenge component of the study (see below). The average ages of the animals within each group were 7.42±4.26 years for the unvaccinated group, 7.38±4.50 years for the BCG-vaccinated group and 6.75±4.02 years for the MtbΔ sigH group, and these were not statistically significant differences ( Supplementary Fig. 6 ). Aerosol procedures for both vaccination and Mtb challenge Animals were both aerosol-vaccinated and challenged with Mtb using the same methodology and equipment configuration. A custom head-only dynamic inhalation system housed within a class III biological safety cabinet was used for this purpose [63] . The use of this inhalation system for aerosol delivery to non human primate (NHP) [63] has been described for numerous studies involving Mtb [20] , [25] , [29] , [32] as well as other agents [64] . Initially, the respective microbial efficiencies of MtbΔ sigH gene mutant and the parental Mtb CDC1551 strains were determined through a series of aerosol-only studies. The microbial efficiencies were used to estimate achievable aerosol doses that could be delivered to each animal using mathematical formula catered to this purpose [65] for both the aerosol vaccination and subsequent challenge experiments. The animal vaccinations (and challenge exposures) were performed singly, and a ‘target’ dose is reported for the group based on prevailing experimental conditions, including individual animal respiratory rate, during each exposure event. Actual individual dose is based on post hoc analysis of active aerosol sampling of the inhalation chamber during the time of each vaccination and bacterial challenge. All aerosol infections were performed in a single day. Clinical procedures including sampling and euthanasia Vaccines were delivered directly to the deep lung via the aerosol route in a manner similar to how the Mtb challenge is administered. Eight weeks post vaccination, each of the three groups was infected via the inhalation route with a target dose of 1,000 CFU of Mtb CDC1551. Samples were collected before vaccination, post vaccination and post infection. For the sake of clarity, results from vaccinated and infected NHPs are reported in two phases: post vaccination, which means after aerosol vaccination with either BCG or MtbΔ sigH , put before challenge with Mtb and post infection (or post challenge), that is, after challenge with Mtb . A tuberculin skin test was performed before vaccination (−2 weeks), post vaccination (3 weeks) and post infection (11 weeks) as previously described by administration of mammalian tuberculin into the right eyelid [20] , [24] , [25] , [29] , [32] , [33] . Thoracic radiographs (CXRs) were acquired 2 weeks before vaccination and at 3, 7, 11 and 14 weeks post vaccination as previously described [20] , [24] , [25] , [29] , [32] , [66] . Briefly, the CXRs were scored by veterinary clinicians in a blinded manner on a subjective scale of 0–4, with a score of 0 denoting normal lung and a score of 4 denoting severe tuberculous pneumonia and pathology. Before vaccination/infection, all 21 animals received a score of 0, as their lungs were perfectly normal at this time. The following subjective scoring system was used: 0 (no pathological involvement); 1 (mild pathological involvement); 2 (moderate pathological involvement); 3 (extensive pathological involvement) and 4 (severe pathological involvement). Blood was drawn before vaccination (−2 weeks) and then weekly thereafter for the performance of complete blood count and serum chemistry [20] , [24] , [25] , [29] , [32] . Blood collected in EDTA tubes (Sarstedt AG & co.) was used for whole-blood flow cytometry using panels described previously [67] . Blood collected in Cell Preparation tubes (Sarstedt AG & co.) was used to isolate PBMC for antigen-specific assays. BAL samples were obtained as previously described, using two washes of 40-ml sterile saline 2 weeks before vaccination and at 3, 7, 11 and 14 weeks [20] , [24] , [25] , [29] , [32] and analysed for CFUs. Necropsy to collect tissues was performed during euthanasia. There were two different reasons for euthanasia. In all 100% (7/7) unvaccinated control animals, as well as ∼ 57% (4/7) of BCG-vaccinated animals, disease progressed to an extent that humane euthanasia was deemed necessary by clinical veterinarians on this team ( Fig. 8h and Supplementary Table 1 ). These humane end points were pre-defined in the animal-use protocol and applied as a measure of reduction of discomfort. The TNPRC Institutional Animal Care and Use Committee approved all animal-related procedures and activities. BCG-vaccinated (43% (3/7)) and MtbΔ sigH -vaccinated (100%) animals were either disease-free or had not progressed to an extent that required humane euthanasia till day 60. Such animals were euthanized for tissue collection via necropsy at that point (between days 60 and 62). At necropsy, lung, spleen and liver tissues were collected and processed as previously described, and CFUs were determined per gram of tissue, using four pooled lung samples per animal, each of which comprised five sections each, thus representing every lung lobe with at least one sample [20] , [24] , [25] , [29] , [32] . A subset of colonies obtained post-challenge necropsy was assayed for resistance to hygromycin to classify them as residual MtbΔ sigH , and subjected to PCR for sigH and esat 6 to classify them as residual MtbΔ sigH and BCG, respectively. No evidence of residual MtbΔ sigH or BCG was found. End point criteria for euthanasia were previously described. Briefly, animals were euthanized if they exhibited four or more of the following: (I) a 2 °F increase in body temperature relative to pre-infection values that persisted for three or more consecutive weeks; (II) a 15% or greater loss in body weight; (III) serum CRP values greater than 10 mg ml −1 for two or more consecutive readings; (IV) CXR values higher than 2; (V) respiratory discomfort resulting in vocalization; (VI) significant-to-complete loss of appetite; and (VII) detectable bacilli in BAL samples. CRP values were included as criteria for euthanasia because CRP is a marker for systemic inflammation that exhibits a high degree of correlation with active TB in macaques [20] , [24] , [25] , [29] , [32] , [33] . Lung pathology at necropsy was determined as described earlier [21] , [26] , [29] , [30] , [38] using stereological principles described by Sharpe et al . [27] . Briefly, lung involvement was quantified by point counting using an overlaid grid with 18.5-mm point spacing. Towards this end, digital images of three systematic random microscopic fields with an original magnification of × 2.5 per slide were employed. At least one sample from each of the four lobes of each lung was used. Intersections representing normal lung included interstitium and air space, while lesions comprised intersections with massive areas of inflammatory cells, haemorrhage, oedema, necrosis or individual to multifocal to lobar granulomas. Differences between completely normal and somewhat inflammed airspace containing localized, small zones of subacute inflammation sans fibrous or cellular encapsulation were not differentiated. Transcriptomics BAL samples were obtained from animals before vaccination (−2 weeks), post vaccination (weeks 3 and 7) and post infection (weeks 11 and 14) as previously described [20] , [24] , [25] , [29] , [32] , [33] , [68] . For stabilization, 8 ml of 100% fetal bovine serum (Invitrogen, Life Sciences) was immediately added to 80 ml of the BAL sample. The sample was centrifuged at 400 r.p.m. for 10 min at 4 °C in an Allegra benchtop centrifuge. The pelleted cells were washed with cold RPMI media (Invitrogen, Life Sciences) and stored at −80 °C until analysis. For transcriptomics, total macaque RNA was isolated from total BAL obtained at the pre-vaccination and the 3 week post-vaccination time points as previously described [30] using an RNAEasy kit (Qiagen), followed by RNA amplification (Ambion MessageAmp). The cDNA derived from the amplified RNA samples from pre-vaccination time points were labelled with Cy3, and samples from the 3-week post-vaccination time point were labelled with Cy5 (Agilent Technologies). Microarray analyses were performed as previously described by assessing the relative expression of transcripts in the Cy5 (experimental)-labelled samples relative to the Cy3(control)-labelled samples, using Agilent 4 × 44 k Rhesus Monkey microarrays [20] , [24] , [25] , [68] . Global impact of expression profiles was analysed using Database for Annotation, Visualization and Integrated Discovery (DAVID) [30] . iBALT Immunofluorescence confocal microscopy was used to measure iBALT as previously described using formalin-fixed, paraffin-embedded tissue [31] , [69] . Flow cytometry Flow cytometry was performed on whole-blood and BAL samples obtained from all 21 animals as previously described [25] , [33] . For T-cell phenotyping, the following antibodies were used: CD3 V500 (1:50, clone SP34-2), CD4 PerCP-Cy5.5 (1:10, clone L200), CD8 PE-TxRed (1:30, clone RPA-T8), CD28 APC (1:5, clone CD28.2), CD69 APC-Cy7 (1:20, clone FN50), CD95 PE-Cy5 (1:5, clone DX2), CD183 AL488 (1:10, clone 1C6/CXCR3), CD184 PE-Cy5 (1:5, clone 12G5), CD195 APC (1:5, clone 3A9), CD197 PE-Cy7 (1:20, clone 3D12), HLA-DR APC-Cy7 (1:75, clone L243) and Ki67 PE-Cy7 (1:50, clone B56) all purchased from BD Biosciences (San Jose, CA, USA). Flow cytometry analyses were conducted by gating first on lymphocytes followed by the elimination of B cells by gating for CD20. The remaining cells were gated for the selection of T cells using CD3, followed by gating into CD3 + CD4 + and CD3 + CD8 + subpopulations. The frequencies of CD4 + and CD8 + T cells expressing activation and homing markers were compared using Ki67, CXCR3, CCR5 and CCR7 (ref. 70 ). The levels of Foxp3 + were determined as a measure of the T reg response. Finally, the extent of CD4 + and CD8 + cells belonging to either T CM or T EM relative to the naive T-cell population were measured using a combination of CD28 and CD95 markers [37] . Antigen-specific immune response PBMCs isolated from whole blood collected from unvaccinated, vaccinated and infected NHPs were stimulated with Mtb cell wall extract (BEI Resources) for the performance of intracellular cytokine staining as previously described, using Mtb cell filtrate protein and cell wall extract for stimulation [57] . In vitro infection of rhesus macaque BMDMs Rh-BMDMs were generated and infected with Mtb CDC1551, the isogenic MtbΔ sigH mutant in this strain, and BCG at an multiplicity of infection of 1:10 as previously described, for 4 h (refs 22 , 46 ). CFUs were measured as described at different time points including 4, 24, 48, 72, 96 and 120 h. CXCL13 expression was measured using DNA microarray [25] and quantitative RT–PCR [22] . The expression of pro-inflammatory mediators TNF-α, IL-1β and IL-6 was measured using real-time RT–PCR as described earlier [22] . The expression of specific chemokines, for example, CXCL9 and CXCL10, was measured using the Cytokine Monkey Magnetic 29-Plex Panel kit from Life-Tech, essentially as described earlier [22] . Statistical analyses Statistical comparisons were performed using one-way or two-way ANOVA in GraphPad Prism with Sidak’s correction for multiple hypotheses. Analysis of transcriptome data was performed using Spotfire DecisionSite [24] , [25] , [68] LOWESS scripts, Ingenuity Pathways Analysis and DAVID as previously described [25] . Specifically, genes with twofold or greater induction in triplicate samples from either vaccination were uploaded to DAVID, and statistically significant accumulation of terms calculated. Accession codes: DNA microarray data have been deposited in the Gene Expression Omnibus under the Accession number GPL10183 . How to cite this article: Kaushal, D. et al . Mucosal vaccination with attenuated Mycobacterium tuberculosis induces strong central memory responses and protects against tuberculosis. Nat. Commun. 6:8533 doi: 10.1038/ncomms9533 (2015).